Chiral recognition and selection during the self-assembly process of protein-mimic macroanions The research on chiral recognition and chiral selection is not only fundamental in resolving the puzzle of homochirality, but also instructive in chiral separation and stereoselective catalysis. Here we report the chiral recognition and chiral selection during the self-assembly process of two enantiomeric wheel-shaped macroanions, [Fe 28 ( μ 3 -O) 8 (Tart) 16 (HCOO) 24 ] 20− (Tart= D - or L -tartaric acid tetra-anion). The enantiomers are observed to remain self-sorted and self-assemble into their individual assemblies in their racemic mixture solution. The addition of chiral co-anions can selectively suppress the self-assembly process of the enantiomeric macroanions, which is further used to separate the two enantiomers from their mixtures on the basis of the size difference between the monomers and the assemblies. We believe that delicate long-range electrostatic interactions could be responsible for such high-level chiral recognition and selection. The homochirality of basic biological molecules such as amino acids and sugars, an intriguing puzzle in modern chemistry, is still not clearly understood [1] , [2] , [3] , [4] , [5] . Current research on the mechanism of homochirality mainly focuses on chiral recognition and chiral selection through studies of chirality transfer and amplification induced by chemical reactions, force fields [3] , [6] , [7] , [8] , [9] , [10] , [11] , [12] , physical properties of solid samples (including crystallization) [13] , [14] , [15] , amino-acid clustering in gas phase [16] , molecular interaction on surfaces [17] , [18] , [19] , [20] and supramolecular assemblies of chiral molecules in bulk and solutions [21] , [22] , [23] , [24] , [25] , [26] , [27] , [28] , [29] , [30] . A few sketchy theories have been developed to explain how homochirality originated, was amplified in macromolecules and supramolecular assemblies and was transmitted to other biomolecules/assemblies during the evolution of life [2] , [31] . This process certainly involves recognition and competition between the enantiomers during their organization into supramolecular structures [32] , [33] . The limitation of stereoselective synthetic technology and the rare examples of the natural biomacromolecule enantiomers make it difficult to study chiral recognition/selection. Through manipulating intermolecular hydrogen bonding and aromatic stacking interactions, Aida and Meijer et al . observed the self-sorted behaviour in the solution of organic enantiomers during their formation of one-dimensional supramolecular structure [27] , [28] , [29] . However, the investigation of physical interactions (for example, electrostatic interaction) and spherical supramolecular assemblies (good analogues of virus capsid) in chiral recognition and selection is still rare. Macroions are soluble ions that are a few nanometres in size; examples include various polyoxometalate molecular clusters, metal–organic nanocages, dendrimers and some biomacromolecules. They exhibit solution behaviour distinct from that associated with simple ions and large colloids [34] , [35] , [36] . When bearing moderate charges, these macroions can strongly attract each other via counterion-mediated interactions and sometimes also hydrogen bonding, forming stable, robust supramolecular assemblies in polar solvents, that is, single-layered, hollow, spherical ‘blackberry’ structures [36] . This self-assembly allows relatively simple building blocks to organize themselves into larger supramolecular structures, a phenomenon that has parallels with the formation of viral capsids (both in morphology and kinetics) [37] . Furthermore, two almost identical macroions remain self-sorted and assemble into homogeneous ‘blackberry’ structures in solutions containing both, demonstrating a high level of self-recognition mimicking biosystems [38] , [39] . Here two inorganic chiral macroions, [Fe 28 ( μ 3 -O) 8 (Tart) 16 (HCOO) 24 ] 20− (Tart= D -(S,S)-(-)-tartaric acid tetra-anion, D-Fe 28 ; Tart= L -(R,R)-(+)-tartaric acid tetra-anion, L-Fe 28 ), are used as simple models, for the first time, to study the role of one type of universal physical interaction, electrostatic interaction, in chiral recognition and selection behaviour of biomolecules in solution. The kinetics study of the self-assembly indicates that the two enantiomers recognize each other and form their individual ‘blackberry’ structures. The addition of chiral co-anions is critical to selectively suppress the self-assembly process of one of the enantiomers. This study provides a new way to experimentally achieve chiral separation. Molecular structures of the chiral macroanions The nano-scaled anionic ferric wheel [Fe 28 ( u 3 -O) 8 (Tart) 16 (HCOO) 24 ] 20− consists of four {Fe 7 } subunits connected by four Tart linkers ( Fig. 1 and Supplementary Figs 1–12 and Supplementary Tables 1–5 ) [40] . If the building units, the Tart ligands, are treated as ‘amino acids’, the Fe 28 cluster can be considered as a protein-mimic molecule involving ‘polymerization’ of 16 such ‘amino acids’ via the connections to Fe 3+ . Therefore, it is straightforward to understand chiral recognition and chiral selection among biomacromolecules from the corresponding studies of Fe 28 chiral clusters. Small-angle X-ray scattering, zeta-potential measurements and structural analysis confirm that Fe 28 clusters preserve their molecular structures in aqueous solution and stay as macroanions with associated counterions around their surface without involving any hydrophobic or intermolecular chemical interactions ( Supplementary Figs 13–17 ). 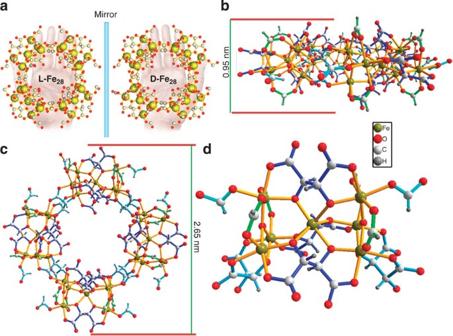Figure 1: Molecular structures of enantiomers of Fe28clusters. (a) Ball–stick representation of molecular structures of enantiomers of Fe28. (b,c) Side and top view of the molecular structures ofL-Fe28(molecular units highlighted in blue are tartaric acid fragments). (d) Ball–stick representation of {Fe7} subunit of the cluster. Colour code of the fragment: blue and teal, two coordination modes of Tart; bright green and turquoise, two coordination modes of methanoate group. Figure 1: Molecular structures of enantiomers of Fe 28 clusters. ( a ) Ball–stick representation of molecular structures of enantiomers of Fe 28 . ( b , c ) Side and top view of the molecular structures of L-Fe 28 (molecular units highlighted in blue are tartaric acid fragments). ( d ) Ball–stick representation of {Fe 7 } subunit of the cluster. Colour code of the fragment: blue and teal, two coordination modes of Tart; bright green and turquoise, two coordination modes of methanoate group. Full size image Chiral recognition between macroanionic enantiomers With the aim of using simple macroions to understand some fundamental processes and features in biological systems, we study the racemic mixture solutions of the Fe 28 enantiomers to determine whether they form homogeneous or heterogeneous ‘blackberry’ structures without any disturbance. With Ba 2+ being counterions, Ba-D-Fe 28 (0.5 mg ml −1 ), Ba-L-Fe 28 (0.5 mg ml −1 ) and their racemic mixture ( D / L =1:1, 0.25 mg ml −1 for each) in water, as monitored by the static light scattering (SLS) technique, all show a slow self-assembly process and reach equilibrium in ∼ 10 days ( Fig. 2a ). The two enantiomers self-assemble at the same speed, as confirmed by time-resolved SLS measurements. Since the self-assembly rate is proportional to the macroionic concentration ( Supplementary Fig. 18 and Supplementary Note 1 ), the time-resolved SLS curve for the mixed solution should be similar to the two individual enantiomeric solutions if no recognition exists between the two enantiomers. However, the rate is much slower in the solution of racemic mixtures and the equilibrium state achieved is at a much lower scattered intensity. This observation implies that the two enantiomers can recognize each other and form their individual assemblies ( Fig. 2c ) [38] . Laser light scattering (LLS) [41] and transmission electron microscopy (TEM) studies of the above three solutions indicate that hollow spherical assemblies of hydrodynamic radius ( R h ) as ca 65±4 nm form during the self-assembly process ( Fig. 2b and Supplementary Figs 19 and 20 ). 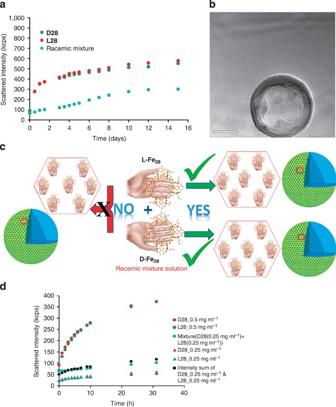Figure 2: Self-recognition behaviour among the enantiomers of Fe28clusters. (a) SLS results ofBa-D-Fe28,Ba-L-Fe28and their racemic mixture solutions. (b) TEM image of the assembly in the aged solution ofBa-D-Fe28(0.5 mg ml-1). Scale bar, 50 nm. (c) Graphical representation of the chiral recognition behaviour. (d) SLS monitoring of different solutions for 31 h. Figure 2: Self-recognition behaviour among the enantiomers of Fe 28 clusters. ( a ) SLS results of Ba-D-Fe 28 , Ba-L-Fe 28 and their racemic mixture solutions. ( b ) TEM image of the assembly in the aged solution of Ba-D-Fe 28 (0.5 mg ml -1 ). Scale bar, 50 nm. ( c ) Graphical representation of the chiral recognition behaviour. ( d ) SLS monitoring of different solutions for 31 h. Full size image The two individual enantiomer solutions (0.5 mg ml −1 ) and their mixtures ( D / L =1:1; 0.25 mg ml −1 for each) were monitored by SLS for the first 31 h after preparation to check whether the lag phase period, known as the dimer/oligomer formation stage, is responsible for the self-recognition behaviour [37] . The first two solutions self-assemble at almost the same rate and much faster than that of the mixed solution, confirming that the self-recognition starts at the early stage of the assembly ( Fig. 2d ). The scattered intensity from the D / L mixed solution (0.25 mg ml −1 each, blue dots in Fig. 2d ) also grows slower than the sum of the scattered intensities of two individual enantiomer solutions at 0.25 mg ml −1 (black dots in Fig. 2d ), indicating that the presence of the other type of monomer seems to negatively impact the assembly process, possibly due to the ineffective collisions among the macroions. The rigid nature of the monomer structure and the high energy barrier for dimer/oligomer formation are expected to be important for the self-recognition. Olson et al . [42] studied the chiral recognition theoretically and suggested that only homochiral oligomers were observed at the beginning and homogeneous assemblies were obtained at the end, which is consistent with our observations. SLS studies on the solutions of another completely different pair of inorganic macroanionic enantiomers {[α-P 2 W 15 O 55 (H 2 O)]Zr 3 (μ 3 -O)(H 2 O)(L-tartH)[α-P 2 W 16 O 59 ]} 15− ( L -CH) and {[α-P 2 W 15 O 55 (H 2 O)]Zr 3 (μ 3 -O)(H 2 O)(D-tartH)[α-P 2 W 16 O 59 ]} 15− ( D -CH) with dimension 2.4 × 1.0 × 0.9 nm 3 (ref. 43 ) and their racemic mixture, respectively, confirm the chiral recognition during the self-assembly process of chiral macroions ( Supplementary Figs 21 and 22 , and Supplementary Note 2 ). Dimers/oligomers are considered as the intermediate state in the self-assembly process [37] . Owing to the morphological compatibility, the formation energy for homo-oligomers might be slightly lower than the hybrid oligomers. This tiny difference will be continuously amplified during the multiple steps of association and it leads to the dominance of homogeneous blackberries over heterogeneous ones. Chiral selection via the introduction of chiral co-anions Small chiral organic molecules (for example, lactic acid) are found to selectively suppress the self-assembly process of the enantiomers of Ba-Fe 28 . As weak acids, lactic acids partially exist as anions in aqueous solution [44] . For Ba-D-Fe 28 and Ba-L-Fe 28 (0.5 mg ml −1 ) in three aqueous solutions containing D -lactic acid (33 μg ml −1 ), L -lactic acid (33 μg ml −1 ) and D / L -lactic acid (16.5 μg ml −1 for each) as chiral buffers, respectively, the D-Fe 28 macroanions are observed to self-assemble rapidly in the solution of L -lactic acid with a short lag phase period (<1 day). However, in the solution of D -lactic acid, the assembly process is slower with a longer lag phase of ∼ 10 days ( Fig. 3a,b and Supplementary Fig. 23 ). The assembly speed of the D-Fe 28 in the buffer of mixed D / L -lactic acids stays in the middle of the above two solutions with a lag phase of ∼ 6 days ( Fig. 3b ). Identically, the assembly speed of L-Fe 28 is the fastest and with the shortest lag phase time (<1 day) in the solution of D -lactic acid, followed by the D / L -lactic acid mixed solution and the L -lactic acid solution ( Fig. 3a,c and Supplementary Fig. 23 ). The explanation for these observations is that D -lactic acid selectively suppresses the self-assembly of D-Fe 28 while L -lactic acid suppresses that of L-Fe 28 . To observe the counter-cations playing a critical role on controlling the assembly of Fe 28 macroanions is expected; however, the current results show that the co-anions (here lactic acids) are also involved in the assembly process. A small preference from the environment can lead to a complete chiral selection during assembly. Similar to the chiral recognition study, the chiral selection was proved to start during the lag phase period of the self-assembly process. The lag phase periods for the solutions of D-Fe 28 and L-Fe 28 (0.5 mg ml −1 ) in the buffer of L -lactic acid (33 μg ml −1 ) were determined as ∼ 50 and ∼ 270 h, respectively ( Fig. 3d ). In the buffer with L -lactic acid, the formation of D-Fe 28 dimers/oligomers at the beginning of the self-assembly is much faster than that of L-Fe 28 . 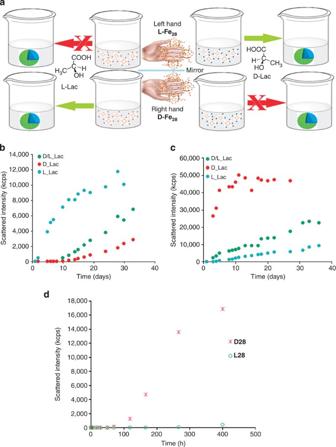Figure 3: Chiral selection during the self-assembly process of Fe28. (a) Graphical representation of the chiral selection experiments by the introduction of lactic acid molecules. (b,c) SLS results ofBa-D-Fe28(0.5 mg ml−1) andBa-L-Fe28(0.5 mg ml−1) in three different buffers, respectively. (d) SLS monitoring of Ba-D-Fe28and Ba-L-Fe28(0.5 mg ml−1) in the buffer ofL-lactic acid (33 μg ml−1) over a period of 400 h. Figure 3: Chiral selection during the self-assembly process of Fe 28 . ( a ) Graphical representation of the chiral selection experiments by the introduction of lactic acid molecules. ( b , c ) SLS results of Ba-D-Fe 28 (0.5 mg ml −1 ) and Ba-L-Fe 28 (0.5 mg ml −1 ) in three different buffers, respectively. ( d ) SLS monitoring of Ba-D-Fe 28 and Ba-L-Fe 28 (0.5 mg ml −1 ) in the buffer of L -lactic acid (33 μg ml −1 ) over a period of 400 h. Full size image Further studies were conducted using the buffers containing other chiral molecules, neutral arabinose and anionic tartaric acid, to determine whether the anionic feature of added chiral organic molecules is critical for the chiral selection. Ba-D-Fe 28 and Ba-L-Fe 28 self-assemble at a similar rate in both D -arabinose and L -arabinose (78 μg ml −1 ) buffers ( Supplementary Fig. 24 ), confirming that no chiral selection can be observed in the buffers of arabinose. However, time-resolved SLS studies on D-Fe 28 and L-Fe 28 in D-(S,S)-(−)- and L -(R,R)-(+)-tartaric acid buffers, respectively, indicate that the self-assembly process of D-Fe 28 can be suppressed by L -tartaric acid in the buffer (31 μg ml −1 ) and that of L-Fe 28 can be suppressed by D -tartaric acid in the buffer (31 μg ml −1 ) ( Supplementary Figs 25 and 26 ). The study with buffers containing three different chiral organic molecules demonstrates the significance of co-anions in chiral selection during the self-assembly process of chiral macroanions ( Supplementary Table 6 ). The chiral selection during the self-assembly process could result from the compatibility between chiral co-anions (lactic acid or tartaric acid) and the chiral microenvironment confined by the macroions. In the lag phase period, discrete macroanionic clusters, surrounded by counterions and loosely by some co-anions, collide with each other to slowly form dimer (or oligomer) structures. It is well known that the counterions mediate the attraction in confined spaces between the clusters, the so-called chiral microenvironment ( Fig. 4a ) [45] . The new results indicate that the loosely associated co-anions are also involved in dimer formation. The compatibility of lactic acid/tartaric acid and the chiral microenvironment determines the rate of self-assembly very likely by affecting both the pre-exponential frequency (reactant encounter probability) as was the activation energy for formation of dimers/oligomers. Experimental results confirm that the D -lactic acid is compatible with the chiral microenvironments of L-Fe 28 , and vice versa . These preferred pairs (for example, D -lactic acid ( L -tartaric acid)/ L-Fe 28 ) very likely have slightly lower activation energies for dimer/oligomer formation, leading to shorter lag phase periods, and consequently more dominant blackberry formation. LLS [41] and TEM measurements indicate that the preferred pairs form larger blackberry structures ( R h ∼ 63±4 nm) than the unpreferred pairs (for example, D -lactic acid/ D-Fe 28 ) do ( R h ∼ 40±2 nm) ( Fig. 4b,c and Supplementary Figs 27 and 28 ). The observation indicates that the macroions with preferred partners interact more strongly with each other in the assembly structures, resulting in a shorter inter-macroionic distance and consequently smaller curvature of the spherical shell, that is, larger blackberry sizes. 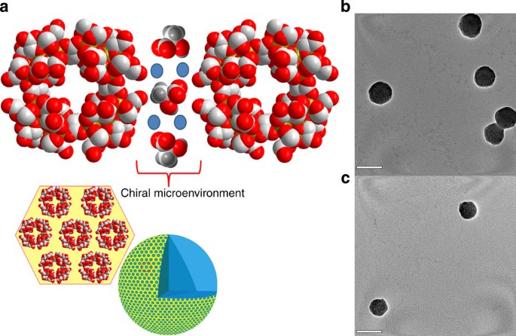Figure 4: The mechanism for chiral selection. (a) Graphical representation of chiral microenvironment confined by two Fe28clusters in their dimeric structure. Colour code of the spheres: yellow, Fe; red, O; blue, Ba2+; light grey, C; dark grey, H. (b,c) TEM images of the assemblies in Ba-D-Fe28(0.5 mg ml−1) and Ba-L-Fe28(0.5 mg ml−1) in the buffer ofL-lactic acid (33 μg ml−1), respectively. Scale bar, 100 nm. Figure 4: The mechanism for chiral selection. ( a ) Graphical representation of chiral microenvironment confined by two Fe 28 clusters in their dimeric structure. Colour code of the spheres: yellow, Fe; red, O; blue, Ba 2+ ; light grey, C; dark grey, H. ( b , c ) TEM images of the assemblies in Ba-D-Fe 28 (0.5 mg ml −1 ) and Ba-L-Fe 28 (0.5 mg ml −1 ) in the buffer of L -lactic acid (33 μg ml −1 ), respectively. Scale bar, 100 nm. Full size image Chiral separation from the enantiomer mixture The individual enantiomers can be separated from their racemic mixtures by the introduction of the chiral anionic molecules due to the synergistic impact of both chiral recognition and chiral selection ( Supplementary Note 3 ). For a racemic mixture of Ba-Fe 28 (0.25 mg ml −1 for each) in the buffer of D -lactic acid (66 μg ml −1 ) after blackberry formation, the enantiomers were easily separated by filter membranes (molecular weight cutoff, 30 kDa). L-Fe 28 macroions self-assemble dominantly, while most D-Fe 28 stay as single clusters ( Fig. 5a,b ). The upper layer solution, expected to contain only large assemblies, shows the signal of L-Fe 28 , while the bottom layer solution, expected to be dominated by monomers, shows the signal of D-Fe 28 ( Fig. 5c–e ). This indicates that the two enantiomers were successfully separated. 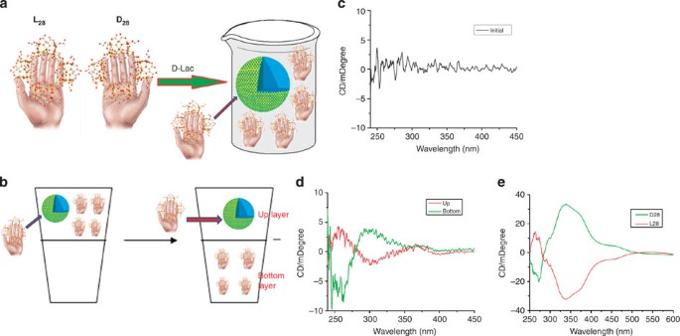Figure 5: Chiral separation from the synergistic effect of chiral recognition and selection. (a) Graphical representation of the self-assembly of the two enantiomers in theD-lactic buffer. (b) Graphical representation of ultrafiltration experiment. (c) CD spectrum of the solution before ultrafiltration. (d) CD spectra of upper layer (red) and bottom layer (green) solutions after ultrafiltration. (e) CD spectra of aqueous solutions of pure Ba-D-Fe28(green) and pure Ba-L-Fe28(red). Figure 5: Chiral separation from the synergistic effect of chiral recognition and selection. ( a ) Graphical representation of the self-assembly of the two enantiomers in the D -lactic buffer. ( b ) Graphical representation of ultrafiltration experiment. ( c ) CD spectrum of the solution before ultrafiltration. ( d ) CD spectra of upper layer (red) and bottom layer (green) solutions after ultrafiltration. ( e ) CD spectra of aqueous solutions of pure Ba-D-Fe 28 (green) and pure Ba-L-Fe 28 (red). Full size image In summary, chiral macroanions demonstrate chiral recognition behaviour by forming homogeneous blackberry structure via long-range electrostatic interactions between the individual enantiomers in their racemic mixture solutions. Adding chiral co-anions suppresses the self-assembly of one enantiomer while maintaining the assembly of the other one. This leads to a natural chiral selection and chiral amplification process, indicating that some environmental preferences can lead to a complete chiral selection. The fact that the relatively simple inorganic macroions exhibit chiral recognition and selection during their assembly process indicates that the related features of biomacromolecules might be due to their macroionic nature via long-range electrostatic interactions. Buffer preparation Solution A was prepared by adding 100 ml of formic acid to 50 g of Ba(OH) 2 ·8H 2 O dissolved in 500 ml water. Solution B was prepared by adding 90 ml of propanoic acid to a solution of 15 g Ca(OH) 2 dissolved in 500 ml water. Synthesis of Ba-L-Fe 28 To 30 ml of solution A , 8 ml of 1 M Fe(NO 3 ) 3 aqueous solution and 0.25 g of L -tartaric acid were added. Another 4.0 g of Ba(OH) 2 ·8H 2 O was added to the mixture solution. The obtained solution was heated to 50 °C with stirring for 3 h. The resulting solution was filtered hot to remove any precipitate and left in a refrigerator at 4 °C for crystallization. A mixture of dark red crystals and chunky crystalline powder started to form after 3 days, and the high-quality dark red crystals were collected by filtration after 10 days (yield 0.68 g dark red crystals; ca 32.5%, based on Fe). One single crystal was submitted to structural analysis by X-ray crystallography and the bulk sample was analysed by elemental analysis. Ba-L-Fe 28 : Ba 10 [Fe 28 ( μ 3 -O) 8 (Tart) 16 (HCOO) 24 ]·47H 2 O. Anal. Calcd (%): Ba, 18.73; Fe, 21.33; Found: Ba, 17.95; Fe, 20.60. Synthesis of Ba-D-Fe 28 To 30 ml of solution A , 8 ml of 1 M Fe(NO 3 ) 3 aqueous solution and 0.25 g of D -tartaric acid were added. Another 4.0 g of Ba(OH) 2 ·8H 2 O was added to the mixture solution. The obtained solution was heated to 50 °C with stirring for 3 h. The resulting solution was filtered hot to remove any precipitate and left in a refrigerator at 4 °C for crystallization. A mixture of dark red crystals and chunky crystalline powder started to form after 3 days, and the high-quality dark red crystals were collected by filtration after 10 days (yield 0.54 g dark red crystals; ca 25.2%, based on Fe). One single crystal was submitted to structural analysis by X-ray crystallography and the bulk sample was analysed by elemental analysis. Ba-D-Fe 28 : Ba 10 [Fe 28 ( μ 3 -O) 8 (Tart) 16 (HCOO) 24 ]·57H 2 O. Anal. Calcd (%): Ba, 18.29; Fe, 20.82; Found: Ba, 18.70; Fe, 20.81. Synthesis of Ca-L-Fe 28 To 30 ml of solution B , 6 ml of 1 M Fe(NO 3 ) 3 aqueous solution and 0.30 g of L -tartaric acid were added. Another 0.45 g of Ca(OH) 2 was added to this solution. The resulting solution was heated to 90 °C with stirring for 2 h then cooled down to room temperature and filtered. Black crystals were obtained after 15 days. Yield, 31% (based on Fe). Ca-L-Fe 28 : Ca 6 H 6 [Fe 28 ( μ 3 -O) 8 (C 4 H 2 O 6 ) 16 (CH 3 CH 2 COO) 22 (H 2 O) 2 ]·76H 2 O. Anal. Calcd (%): Ca, 3.30; Fe, 21.46; Found: Ca, 3.15; Fe, 20.47. Synthesis of Ca-D-Fe 28 To 30 ml of solution B , 6 ml of 1 M Fe(NO 3 ) 3 aqueous solution and 0.30 g of D -tartaric acid were added. Another 0.45 g of Ca(OH) 2 was added to this solution. The resulting solution was heated to 90 °C with stirring for 2 h then cooled down to room temperature and filtered. Black crystals were obtained after 3 days. Yield, 28% (based on Fe). Ca-D-Fe 28 : Ca 6 H 6 [Fe 28 ( μ 3 -O) 8 (C 4 H 2 O 6 ) 16 (CH 3 CH 2 COO) 22 (H 2 O) 2 ]·76H 2 O. Anal. Calcd (%): Ca, 3.30; Fe, 21.46; Found: Ca, 3.06; Fe, 20.27. Static light scattering The solutions for light scattering testing were prepared by dissolving the solid samples in D.I. water with sonication and dialysed against pure D.I. water to remove the extra counterion salts with a 1K dialysis membrane overnight. The resulting solution was transferred in a syringe and pushed to pass through 450 nm filters and into 20 ml glass vials. A commercial Brookhaven Instrument LLS spectrometer equipped with a solid-state laser operating at 532 nm was used for measurement of both SLS and DLS. SLS experiments were performed at scattering angles ( θ ) between 20° and 100°, at 2° intervals. However, due to the large fluctuations in scattered intensities at low scattering angles, data from 20° to 40° in the final analysis were removed. Derived from Rayleigh–Gans–Debye equation [46] , partial Zimm plot was used to analyse the SLS data to obtain the radius of gyration ( R g ). The partial Zimm plot stems from the following approximation: 1/ I = C (1+ R g 2 / q 2 /3). Here R g is determined from the slope and the intercept of a plot of 1/ I versus q 2 . Dynamic light scattering DLS measures the intensity–intensity time correlation function by means of a BI-9000AT multi-channel digital correlator. The field correlation function | g (1) ( τ )| was analysed by the constrained regularized CONTIN method [41] to yield information on the distribution of the characteristic linewidth Γ from | g (1) ( τ )|=∫ G (Γ) e −Γ τ dΓ. The normalized distribution function of the characteristic linewidth, G (Γ), so obtained, can be used to determine an average apparent translational diffusion coefficient, D app =Γ/ q 2 . The hydrodynamic radius R h is related to D via the Stokes–Einstein equation: R h =k T /(6 πηD ) where k is the Boltzmann constant and η the viscosity of the solvent at temperature T . From DLS measurements, we can obtain the particle size distribution in solution from a plot of Γ G (Γ) versus R h . The R h of the particles is obtained by extrapolating R h,app to zero scattering angle. CD spectrum The solution samples were put in a 1-cm cuvette and the solutions were diluted by D.I. water until the HT in the whole wavelength range is <800 mV. The solutions with appropriate concentrations were scanned five times from 600 to 220 nm and the resulting data were averaged after subtracting the baseline of pure solvent (water). Ultrafiltration Ultrafiltration was performed using Macrosep Advance Centrifugal Device (30 K MWCO) to separate blackberry structures and discrete molecular clusters. A sample solution was poured into the device and the device is rotated at a speed of 4,000 g for 50 min. The upper layer and bottom layer were collected for CD spectrum testing. The racemic mixture solution with D -lactic acid was filtered 20 days after its preparation. Several drops of acetic acid were used to help dissolve the red solid on the filter membrane; this redissolved material was combined with the upper layer solution. The X-ray crystallographic coordinates for structures reported in this study have been deposited at the Cambridge Crystallographic Data Centre (CCDC) under deposition numbers 1044500–1044503. These data can be obtained free of charge from The CCDC via http://www.ccdc.cam.ac.uk/data_request/cif . How to cite this article: Yin, P. et al . Chiral recognition and selection during the self-assembly process of protein-mimic macroanions. Nat. Commun. 6:6475; doi: 10.1038/ncomms7475 (2015).